A quantum diffractor for thermal flux Macroscopic phase coherence between weakly coupled superconductors leads to peculiar interference phenomena. Among these, magnetic flux-driven diffraction might be produced, in full analogy to light diffraction through a rectangular slit. This can be experimentally revealed by the electric current and, notably, also by the heat current transmitted through the circuit. The former was observed more than 50 years ago and represented the first experimental evidence of the phase-coherent nature of the Josephson effect, whereas the second one was still lacking. Here we demonstrate the existence of heat diffraction by measuring the modulation of the electronic temperature of a small metallic electrode nearby-contacted to a thermally biased short Josephson junction subjected to an in-plane magnetic field. The observed temperature dependence exhibits symmetry under magnetic flux reversal, and clear resemblance with a Fraunhofer-like modulation pattern. Our approach, joined to widespread methods for phase-biasing superconducting circuits, might represent an effective tool for controlling the thermal flux in nanoscale devices. The first evidence of the d.c. Josephson [1] effect dates back to 1963 when J. S. Rowell measured the diffraction pattern of the critical current flowing through a single superconducting tunnel junction subjected to an in-plane magnetic field [2] . Interference of Josephson currents through two tunnel junctions connected in parallel was achieved 1 year later, leading to the first ever superconducting quantum interferometer [3] . The latter, together with Rowell’s observations, constituted the unequivocal demonstration of the Josephson supercurrent–phase relation. Yet, the Josephson effect has further profound implications going well beyond electrical transport, as the phase of the Cooper pair condensate is encoded in the wave functions of the un-paired Bogoliubov quasiparticles that transport thermal energy as well as electrical charge [4] , [5] , [6] , [7] Here we report the first realization of Fraunhofer diffraction for thermal currents [8] . Specifically, thermal diffraction manifests itself with a modulation of the electron temperature in a small metallic electrode nearby contacted to a thermally biased Josephson junction (JJ) when sweeping the magnetic flux Φ. Remarkably, the observed temperature dependence exhibits symmetry under Φ reversal and a clear reminiscence with a Fraunhofer-like modulation pattern, as expected fingerprints for a quantum diffraction phenomenon. Our results confirm a recent prediction of heat transport [8] and, joined with double-junction heat interferometry demonstrated in ref. 6 , exemplify the complementary proof of the existence of phase-dependent thermal currents in Josephson-coupled superconductors. This approach combined with well-known methods for phase-biasing superconducting circuits provides with a novel tool for control of the heat flux at the nanoscale [9] , [10] . Thermal diffraction Both electric and thermal quantum diffraction may arise in a solid state structure by virtue of the Josephson effect. What these phenomena share in common is phase coherence of either supercurrent or thermal flux flowing through a JJ. To illustrate this, let us assume an ideal rectangular tunnel JJ composed of two superconductors, S 1 and S 2 , separated by a thin insulating layer under the influence of an in-plane magnetic field H . If an electric current I is allowed to flow through the junction, diffraction manifests as the archetypal Fraunhofer interference pattern of the critical current I c (see Fig. 1a ) [2] . By contrast, if the junction is electrically open but a temperature gradient is applied so that S 1 is set at temperature T 1 while S 2 resides at T 2 , a stationary heat current will develop flowing from S 1 to S 2 (see Fig. 1b ). As predicted in ref. 8 the latter will reflect the consequences of quantum diffraction in full similarity with the electric case. In particular, in analogy with Equation (1) of ref. 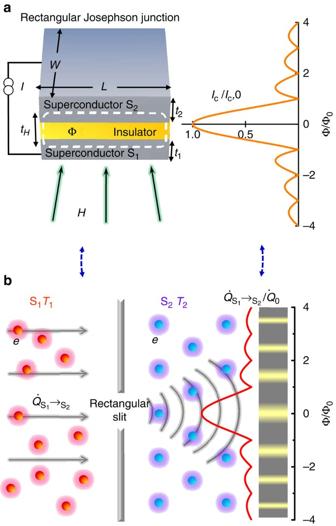Figure 1: Electric versus thermal quantum diffraction through a rectangular slit. (a) The amplitudeIcof the critical current flowing through a rectangular Josephson junction composed of two superconductors, S1and S2, separated by a thin insulating layer displays the archetypal Fraunhofer interference pattern as the magnetic flux Φ threading the junction is varied under an in-plane sweeping magnetic fieldH. (b) Analogously, when the two superconductors are kept at different temperatures,T1>T2, the resulting heat currentflowing through the junction shows fingerprints of phase coherence. This is reflected, similarly, in a Fraunhofer-like modulation ofwith Φ. Both phenomena occur in full analogy to light diffraction through a rectangular slit.Ic,0anddenote the critical and maximum thermal current at zero magnetic field, respectively, whereas Φ0is the magnetic flux quantum andIthe total current flowing through the JJ.L,W,t1andt2denote the junction's main geometrical dimensions andtHis the effective magnetic thickness defined in the text. 6 , is given by [8] Figure 1: Electric versus thermal quantum diffraction through a rectangular slit. ( a ) The amplitude I c of the critical current flowing through a rectangular Josephson junction composed of two superconductors, S 1 and S 2 , separated by a thin insulating layer displays the archetypal Fraunhofer interference pattern as the magnetic flux Φ threading the junction is varied under an in-plane sweeping magnetic field H . ( b ) Analogously, when the two superconductors are kept at different temperatures, T 1 > T 2 , the resulting heat current flowing through the junction shows fingerprints of phase coherence. This is reflected, similarly, in a Fraunhofer-like modulation of with Φ. Both phenomena occur in full analogy to light diffraction through a rectangular slit. I c,0 and denote the critical and maximum thermal current at zero magnetic field, respectively, whereas Φ 0 is the magnetic flux quantum and I the total current flowing through the JJ. L , W , t 1 and t 2 denote the junction's main geometrical dimensions and t H is the effective magnetic thickness defined in the text. Full size image where Φ 0 =2 × 10 −15 Wb is the flux quantum. According to Equation (1), consists of a Fraunhofer-like diffraction pattern (that is, the term containing the sine cardinal function) superimposed on top of a magnetic flux-independent heat current. In particular, will display minima for integer values of Φ 0 as the critical supercurrent does. The first term on the rhs of Equation (1) describes the heat current carried by electrons [11] , where R J is the normal-state resistance of the JJ, is the Bardeen–Cooper–Schrieffer-normalized density of states in the superconductors [12] , f ( T i )=tan h( ε /2 k B T i ), Δ i ( T i ) is the temperature-dependent energy gap of superconductor S i with i =1,2, Θ( x ) is the Heaviside step function, k B is the Boltzmann constant and e is the electron charge. The second term on the rhs of Equation (1) is unique to weakly coupled superconductors and arises from energy-carrying processes involving tunnelling of Cooper pairs, which leads to its peculiar Φ dependence [4] , [13] , [14] , [15] . In particular, where . For small temperature differences δ T = T 1 − T 2 << T =( T 1 + T 2 )/2, the total heat current flowing through the JJ can be written as , where the electron thermal conductance is defined as For identical superconductors, so that Δ 1,2 =Δ, in the low temperature limit k B T <<0 and for Φ=0, we can derive the following approximate analytical expression for , which shows that the total heat current flowing through the junction is exponentially small at low temperature. Device structure A Josephson thermal diffractor (in the following denoted as device A) has been fabricated by electron beam lithography and four-angle shadow mask evaporation of aluminium (Al) and aluminium doped with manganese impurities (Al 0.98 Mn 0.02 ). The former constitutes the superconducting electrodes with critical temperature ≈1.3 K whereas the latter is a normal metal. The device core consists of an extended rectangular JJ made of two tunnel-connected Al electrodes, S 1 and S 2 , with R J ≈870 Ω (see Fig. 2a ). The junction’s geometrical dimensions, defined in Fig. 1a , are L ≈9 μm, W ≈0.3 μm, t 1 ≈30 nm and t 2 ≈80 nm. H is applied in the junction plane and is perpendicular to its largest lateral dimension, that is, L . An extra aluminium probe S 3 is used to current bias the main JJ for preliminary electric characterization. S 3 is connected to S 1 through a bias JJ with normal-state resistance R bias ≈430 Ω placed in orthogonal direction with respect to the main JJ so to be only marginally influenced by H . Heat transport through the structure, on the other hand, is investigated, thanks to two normal metal source and drain Al 0.98 Mn 0.02 electrodes tunnel connected to S 1 while keeping both JJs electrically open. The electronic temperature in the source ( T src ) and in the drain ( T dr ) is experimentally controlled and measured, thanks to a number of normal metal–insulator–superconductor (NIS) probes serving as heaters and thermometers [16] , [17] . Source and drain tunnel junctions have normal-state resistance R s ≈ R d ≈3.5 kΩ whereas each NIS probe exhibits ~20 kΩ on the average. 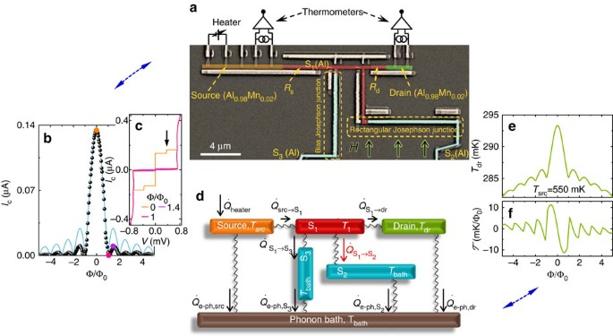Figure 2: The Josephson thermal quantum diffractor. (a) Pseudo-colour scanning electron micrograph of device A. The quantum diffractor for thermal currents is realized by means of a rectangular Josephson tunnel junction made of two Al superconducting electrodes. The first one (S1) is tunnel coupled to two source and drain normal metal electrodes (realized with Al0.98Mn0.02), enabling Joule heating and thermometry.RsandRdare the corresponding normal-state resistances. The second one (S2) extends into a large bonding pad and is kept open during the heat diffraction experiment. The electric characterization of the device is performed through an extra Al probe (S3) tunnel connected to S1through a bias JJ.His the in-plane applied magnetic field. (b) Experimental magnetic diffraction pattern of the critical currentIc(scatter) of the rectangular JJ of device A. Solid line is the theoretical calculation for an ideal rectangular junction. (c) Selected current (I) versus voltage (V) curves corresponding to different Φ values indicated by dots of the same colour inb. Curves inb,cwere measured at 240 mK through the S3–S1–S2series connection. (d) Thermal model accounting for the main heat exchange sources present in the device. For clarity, each box is coloured as its corresponding electrode ina. Electrons in the source are intentionally heated up toTsrcby an injected Joule power,. Electrons in S1residing atT1exchange heat with those in the source at power, at powerandwith electrons in S2and S3, respectively, and at powerwith electrons in the drain. Finally, electrons in the whole structure exchange energy with lattice phonons residing atTbathat power, wherej=src, S2, S3and dr. S2and S3are assumed to reside at the bath temperature (Tbath) owing to their large volume. Arrows indicate the heat flow directions forTsrc>T1>Tdr>Tbath. (e) Electronic temperature of drain electrode (Tdr) versus Φ calculated using the thermal model described indand assumingTsrc=550 mK andTbath=240 mK. Diffraction of thermal currents manifests itself with a peculiar function forTdr, which is symmetric under Φ reversal. (f) Flux-to-temperature transfer coefficient, =∂Tdr/∂Φ, calculated for the same conditions as ine. Figure 2: The Josephson thermal quantum diffractor. ( a ) Pseudo-colour scanning electron micrograph of device A. The quantum diffractor for thermal currents is realized by means of a rectangular Josephson tunnel junction made of two Al superconducting electrodes. The first one (S 1 ) is tunnel coupled to two source and drain normal metal electrodes (realized with Al 0.98 Mn 0.02 ), enabling Joule heating and thermometry. R s and R d are the corresponding normal-state resistances. The second one (S 2 ) extends into a large bonding pad and is kept open during the heat diffraction experiment. The electric characterization of the device is performed through an extra Al probe (S 3 ) tunnel connected to S 1 through a bias JJ. H is the in-plane applied magnetic field. ( b ) Experimental magnetic diffraction pattern of the critical current I c (scatter) of the rectangular JJ of device A. Solid line is the theoretical calculation for an ideal rectangular junction. ( c ) Selected current ( I ) versus voltage ( V ) curves corresponding to different Φ values indicated by dots of the same colour in b . Curves in b , c were measured at 240 mK through the S 3 –S 1 –S 2 series connection. ( d ) Thermal model accounting for the main heat exchange sources present in the device. For clarity, each box is coloured as its corresponding electrode in a . Electrons in the source are intentionally heated up to T src by an injected Joule power, . Electrons in S 1 residing at T 1 exchange heat with those in the source at power , at power and with electrons in S 2 and S 3 , respectively, and at power with electrons in the drain. Finally, electrons in the whole structure exchange energy with lattice phonons residing at T bath at power , where j =src, S 2 , S 3 and dr. S 2 and S 3 are assumed to reside at the bath temperature ( T bath ) owing to their large volume. Arrows indicate the heat flow directions for T src > T 1 > T dr > T bath . ( e ) Electronic temperature of drain electrode ( T dr ) versus Φ calculated using the thermal model described in d and assuming T src =550 mK and T bath =240 mK. Diffraction of thermal currents manifests itself with a peculiar function for T dr , which is symmetric under Φ reversal. ( f ) Flux-to-temperature transfer coefficient, =∂ T dr /∂Φ, calculated for the same conditions as in e . Full size image Low-temperature measurements Quantum diffraction of the electric Josephson current is realized first. The resulting experimental I c versus Φ modulation is shown in Fig. 2b along with the theoretical Fraunhofer diffraction pattern [12] , [18] . I c is an even function of Φ attaining a maximum value of ≈140 nA at Φ=0 and nulling at integer values of Φ 0 , as expected for a rectangular JJ. Differences in the lobes’ amplitude between these curves might reflect non-homogeneous distribution of the supercurrent in the JJ [18] . These data allow to extract the effective magnetic thickness t H of the junction defined by the condition Φ= μ 0 HLt H =Φ 0 , where μ 0 is the vacuum permeability (see Fig. 1a ). From the experimental magnetic field period H ≈40 Oe, we get t H ≈57 nm in good agreement with 59 nm obtained from geometrical considerations [19] . We note that lateral dimensions of the JJs are much smaller than the Josephson penetration depth, ~1 mm, therefore providing the frame of the short junction limit [18] . In such a case, the self-field generated by the Josephson current in the junctions is negligible in comparison with H (ref. 8 ). Data in Fig. 2b are obtained from the zero-voltage steps in the current ( I )–voltage ( V ) characteristics measured through the series connection of the two JJs (see Fig. 2c ). Furthermore, dissipationless electric transport through the main JJ is guaranteed since R bias < R J , leading to a larger critical current in the bias JJ [12] . The ensuing transition of the latter to the dissipative regime is confirmed by the presence of a second switching step at finite voltage in the I – V characteristics (see black arrow in Fig. 2c ). On the other hand, quantum diffraction of thermal currents is realized as follows. A thermal gradient is established by heating intentionally the source’s electrons up to a fixed temperature T src , leading to an increase in the electronic temperature of S 1 up to T 1 > T bath . This is possible since S 1 is a superconducting electrode with small volume ( μm 3 ), allowing for its electrons to be marginally coupled to the lattice phonons at low temperatures [20] . By contrast, S 2 and S 3 are strongly thermalized at T bath stemming from their large volume (~10 4 μm 3 ) [20] . Under these circumstances, T dr is mainly determined by the temperature T 1 in S 1 , which is affected by the heat flux . Therefore, T dr can be used to assess the occurrence of thermal diffraction in the main JJ as H is swept. Insight into this phenomenon can be gained with the help of the thermal model described in Fig. 2d . T 1 and T dr can be calculated for each T src and T bath fixed in the experiment by solving the following system of two non-linear integral thermal-balance equations (see Methods for further details). The latter accounts for the main heat exchange mechanisms occurring in S 1 and drain, respectively, In writing equation (6), we neglect the electron–phonon heat exchange in S 1 since it is much smaller than that existing in the drain electrode, (refs 16 , 20 , 21 ). Heat transport mediated by photons and pure phonon heat current is neglected as well [22] , [23] . In the former case, poor impedance matching with the electromagnetic environment makes indeed thermal transport occurring through the photonic channel vanishing at the investigated bath temperatures [23] , [24] , [25] . As an example, Φ modulation of T dr is calculated at T bath =240 mK using the structure’s parameters for T src =550 mK. The resulting curve is shown in Fig. 2e . Notably, the existence of thermal diffraction leads to a non-monotonic function for the temperature symmetric with respect to Φ reversal, which is maximized at Φ=0, and is suppressed by increasing the magnetic flux. In addition, T dr (Φ) displays minima exactly at integer values of Φ 0 in close resemblance with a Fraunhofer-like diffraction pattern. Figure 2f , on the other hand, shows the corresponding magnetic flux-to-temperature transfer coefficient, =∂ T dr /∂Φ. We stress that the expected temperature modulation arises solely from the combined action of a thermal bias across the JJ and the existence of diffraction of the heat current. Thermal diffraction measurements are performed first at the base temperature of a 3 He refrigerator, that is, T bath ≈240 mK. NIS thermometers in both source and drain electrodes have been calibrated against the cryostat temperature to provide an accurate measure of T src and T dr from the refrigerator base temperature up to ~1 K. Electron thermometry is performed by current-biasing source and drain superconductor–insulator–NIS (SINIS) junctions with 30 and 70 pA, respectively, so as to marginally affect the thermal balance in these electrodes [16] . Source heating, on the other hand, is obtained by delivering a power in the range of ~2–100 pW. The results from SINIS thermometry are then averaged over 30 magnetic field sweeps to accurately measure the dependence of drain electrode temperature on the applied magnetic flux. T dr (Φ) is recorded for different values of T src ranging between ~400 and 800 mK and the resulting curves are plotted in Fig. 3a . The average value of T dr increases as T src is raised up, stemming from a larger heat flow induced in the structure. What is more compelling is the peculiar dependence of T dr on Φ, which consists of a sizable peak centred at Φ=0, surrounded by smaller side lobes preserving symmetry with respect to Φ reversal. These results are in good resemblance with the theoretical prediction (see Fig. 2e ), therefore pointing to the occurrence of quantum diffraction of the thermal flux. This is further proved in Fig. 3b where a few selected T dr (Φ) curves are plotted along with the theoretical expectations (black lines) calculated using the above-described thermal model. 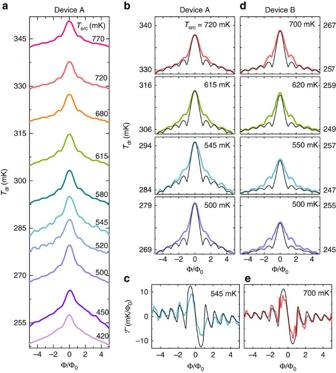Figure 3: Thermal diffraction at 240 mK bath temperature. (a) Gradual increase of the experimentalTdrversus Φ characteristics measured at growingTsrcandTbath=240 mK for device A. Notably,Tdris an even function of Φ showing a well-defined central lobe surrounded by lumps in the amplitude, which decrease as |Φ| increases, in clear resemblance with a Fraunhofer-like diffraction pattern. The amplitude of the central lobe increases initially asTsrcis raised, decreasing slightly at higherTsrc.b,dshow a few experimentalTdrversus Φ temperature curves (colour lines) measured at selected values ofTsrcfor device A and B, respectively. The latter is nominally identical in dimensions to sample A and characterized byRJ≈580 Ω,Rbias≈480 Ω,Rs≈9.5 kΩ,Rd≈14 kΩ and magnetic flux periodH≈37 Oe. The vertical scale in each panel is 13 mK. Remarkably,Tdrexhibits minima at integer multiples of Φ0just as the corresponding experimental critical supercurrent diffraction patterns. Black lines are the theoretical temperature curves obtained using the thermal model described inFig. 2d.c,edisplay the numerically calculated derivative with respect to magnetic flux of the experimentalTdr(Φ) temperature curves at two selected values ofTsrc(coloured lines) and the corresponding calculated theoretical flux-to-temperature transfer functions (black lines) for device A and B, respectively. Figure 3c shows the experimental and theoretical flux-to-temperature transfer coefficient at T src =545 mK. Although rather simplified, our model provides a reasonable qualitative agreement with the experiment, and describes the overall T dr (Φ) modulation shape as well as the exact position of drain temperature minima. In addition, temperature diffraction measurements have been also performed using a similar sample, denoted as device B, leading to comparable results. To illustrate this, Fig. 3d shows a few selected T dr (Φ) characteristics along with the corresponding computed ones. The experimental and theoretical (Φ) traces for device B at T src =700 mK are plotted in Fig. 3e . It is worthwhile to recall that the observed thermal diffraction occurs in the absence of any electric current flowing through the JJs. Figure 3: Thermal diffraction at 240 mK bath temperature. ( a ) Gradual increase of the experimental T dr versus Φ characteristics measured at growing T src and T bath =240 mK for device A. Notably, T dr is an even function of Φ showing a well-defined central lobe surrounded by lumps in the amplitude, which decrease as |Φ| increases, in clear resemblance with a Fraunhofer-like diffraction pattern. The amplitude of the central lobe increases initially as T src is raised, decreasing slightly at higher T src . b , d show a few experimental T dr versus Φ temperature curves (colour lines) measured at selected values of T src for device A and B, respectively. The latter is nominally identical in dimensions to sample A and characterized by R J ≈580 Ω, R bias ≈480 Ω, R s ≈9.5 kΩ, R d ≈14 kΩ and magnetic flux period H ≈37 Oe. The vertical scale in each panel is 13 mK. Remarkably, T dr exhibits minima at integer multiples of Φ 0 just as the corresponding experimental critical supercurrent diffraction patterns. Black lines are the theoretical temperature curves obtained using the thermal model described in Fig. 2d . c , e display the numerically calculated derivative with respect to magnetic flux of the experimental T dr (Φ) temperature curves at two selected values of T src (coloured lines) and the corresponding calculated theoretical flux-to-temperature transfer functions (black lines) for device A and B, respectively. Full size image The robustness of the T dr (Φ) modulation against an increasing bath temperature is shown in Fig. 4a . This leads, on the one hand, to an average enhancement of T dr stemming from a increased total thermal flux through the structure. On the other hand, the amplitude of the modulation decreases and the side lobes fade out as T bath is raised up. This behaviour is emphasized by plotting the T dr (Φ) curves obtained at different T bath after subtraction of an offset (see Fig. 4b ). A sizable central lobe is still clearly visible also for T >400 mK but only for considerably higher source temperatures. The same picture is confirmed by inspecting the corresponding (Φ) transfer functions (see Fig. 4c ). The visibility of the temperature modulation is somewhat degraded for T bath exceeding 450 mK, which can be ascribed to both a reduced temperature biasing across the JJs and enhanced electron–phonon coupling in drain electrode at high T bath (ref. 16 ). 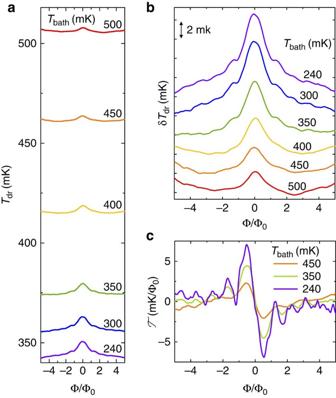Figure 4: Thermal diffraction at several bath temperatures. (a) ExperimentalTdrversus Φ characteristics measured at differentTbathfor device A. From bottom to top, the data were taken atTsrc=770, 780, 880, 885, 920 and 975 mK, respectively. The same curves are offset on the vertical scale and plotted in panel (b) to emphasize differences between them. AsTbathis raised up, the lobes are clearly smeared while the symmetry under Φ reversal is preserved.Tdrmodulation fades out forTbath≳500 mK. The full temperature range is 20 mK, and the vertical division corresponds to 2 mK. (c) Numerically calculated derivative of the experimental drain temperature with respect to magnetic flux versus Φ traces for three selected values ofTbath. Figure 4: Thermal diffraction at several bath temperatures. ( a ) Experimental T dr versus Φ characteristics measured at different T bath for device A. From bottom to top, the data were taken at T src =770, 780, 880, 885, 920 and 975 mK, respectively. The same curves are offset on the vertical scale and plotted in panel ( b ) to emphasize differences between them. As T bath is raised up, the lobes are clearly smeared while the symmetry under Φ reversal is preserved. T dr modulation fades out for T bath ≳ 500 mK. The full temperature range is 20 mK, and the vertical division corresponds to 2 mK. ( c ) Numerically calculated derivative of the experimental drain temperature with respect to magnetic flux versus Φ traces for three selected values of T bath . Full size image A Fraunhofer diffractor for thermal flux has been experimentally realized with a Josephson tunnel junction-based device. Our results confirm a breaking new prediction [8] on phase-coherent heat transport and pave the way for the investigation of more exotic junction geometries [18] , [26] , [27] . These might provide tunable temperature diffraction patterns and should represent a powerful tool for tailoring and managing heat currents at the nanoscale [8] , [29] , [30] , [31] . Besides offering insight into energy transport in quantum nanosystems, our experimental findings set the complementary demonstration of the ‘thermal’ Josephson effect in weakly coupled superconductors, similarly to what it was done 50 years ago for its ‘electric’ counterpart. Sample fabrication and experimental details Device A and B are nominally identical and have been fabricated onto an oxidized Si wafer by e-beam lithography of a suspended resist mask and four-angle shadow mask ultra high vacuum evaporation of metals. The samples are first tilted at 32° to deposit a 15-nm-thick Al 0.98 Mn 0.02 layer, forming source and drain electrodes, and then are exposed to 950 mTorr of O 2 for 5 min, defining the heater, thermometers, source and drain tunnel barriers. A 20-nm-thick Al layer is then deposited by tilting the sample at −49° and, subsequently, a second 30-nm-thick Al layer is evaporated at 32° perpendicularly with respect to the previous directions. These two layers define the S 1 electrode and the superconducting probes of the NIS junctions. A second oxidation process follows at 1.5 Torr for 5 min to form the JJ tunnel barriers. Finally, a 80-nm-thick Al layer is evaporated at 0° to define the S 2 and S 3 electrodes. Magnetoelectric measurements are performed with conventional room temperature preamplifiers. SINIS thermometers are current biased through battery-powered floating sources whereas the heater operates on voltage biasing within 0.5–2 mV. In addition, throughout our measurements we checked that the thermometers response is unaffected by the applied magnetic field. Thermal model In our thermal model (see Equation (6)), and where Φ bias denotes the magnetic flux experienced by the bias JJ, and α and β are the two fitting parameters. Furthermore, and with 3 ( ε , T 3 )= 2 ( ε , T 2 ), 3 ( ε , T 3 )= 2 ( ε , T 2 ) and f ( T 3 )= f ( T 2 ). On the other hand, where f ( T src(dr) )=tan h( ε /2 k B T src(dr) ). Finally, where Σ≈4 × 10 9 WK −6 m −3 is the electron–phonon coupling constant of Al 0.98 Mn 0.02 experimentally measured for our samples [21] , [28] and m 3 is drain volume. To account for the experimental H misalignment, Φ bias ~Φ/15 has been used, which leads to the peculiar ellipsoidal shape of the T dr (Φ) curves. A quantitative agreement between theory and experiment (see Fig. 3 ) can be achieved only by varying α and β between 0.1 and 1. The observed deviations might be ascribed to the presence of nonidealities in the junctions, leading to possible Andreev reflection-dominated heat transport channels [15] , and to a non-homogeneous heat current distribution along the structure. How to cite this article: Martínez-Pérez, M. J. & Giazotto, F. A quantum diffractor for thermal flux. Nat. Commun. 5:3579 doi: 10.1038/ncomms4579 (2014).